Formation of nanodiamonds at near-ambient conditions via microplasma dissociation of ethanol vapour Clusters of diamond-phase carbon, known as nanodiamonds, exhibit novel mechanical, optical and biological properties that have elicited interest for a wide range of technological applications. Although diamond is predicted to be more stable than graphite at the nanoscale, extreme environments are typically used to produce nanodiamonds. Here we show that nanodiamonds can be stably formed in the gas phase at atmospheric pressure and neutral gas temperatures <100 °C by dissociation of ethanol vapour in a novel microplasma process. Addition of hydrogen gas to the process allows in flight purification by selective etching of the non-diamond carbon and stabilization of the nanodiamonds. The nanodiamond particles are predominantly between 2 and 5 nm in diameter, and exhibit cubic diamond, n -diamond and lonsdaleite crystal structures, similar to nanodiamonds recovered from meteoritic residues. These results may help explain the origin of nanodiamonds in the cosmos, and offer a simple and inexpensive route for the production of high-purity nanodiamonds. Carbon exists as a variety of different forms at the bulk and nano scale including graphite, diamond, fullerenes, carbon nanotubes, graphene and nanodiamonds. Graphitic carbon is known to be the most stable form of bulk carbon at ambient temperature and pressure, with high pressures and high temperatures typically required to convert non-diamond phases to diamond [1] , [2] . Atomistic models have predicted that at the nanoscale, hydrogen-terminated tetrahedral hydrocarbons, precursors to diamond phases, are thermodynamically more stable than polycylic aromatics, precursors to graphitic phases, with a transition in the phase stability occurring at ~3 nm (ref. 3 ). This idea supports the existence of naturally formed diamond clusters, referred to as nanodiamonds, in petroleum [4] , interstellar dust [5] and candle flames, [6] all presumably formed at pressures and/or temperatures outside the stability field of bulk diamond. Nanodiamonds have been synthesized for research by several methods including detonation of carbon-containing explosives [7] , [8] and plasma-enhanced chemical vapour deposition (PECVD) [9] . Despite the predicted stability of nanodiamonds, these processes require high pressure and/or high temperature and produce mixtures of non-diamond and diamond phases [10] . Detonation synthesis is carried out at extremely high pressures and temperatures and produces soot containing large quantities of graphitic carbon in addition to the diamond phase [7] . PECVD produces films of amorphous carbon (a-C) with nanodiamonds embedded at the grain boundaries by deposition at high temperatures [9] . Alternatively, it is known that nanoparticles can be homogeneously nucleated in a plasma process [11] , which has the potential to produce nanodiamonds at significantly lower pressures and temperatures and higher purities. However, this approach has thus far been limited to non-diamond carbon [12] and larger diamond particles (~0.1 μm) [13] , [14] . Here we report the synthesis of nanodiamonds at near-ambient conditions using a novel continuous atmospheric pressure, microscale plasma (microplasma) process. Particles are homogeneously nucleated by dissociating ethanol vapour and rapidly quenched with reaction times <1 ms to limit the size of the particles to the nanometre-size regime. By adding H 2 gas, the non-diamond phase is etched and the diamond phase is stabilized, leading to a highly purified as-grown nanodiamond product. The particles exhibit a uniform diameter of ca. 3.0 nm consistent with theoretical predictions [3] , [15] , and cubic diamond, lonsdaleite and the less frequently observed n -diamond phases similar to presolar nanodiamonds recovered from meteorites [16] . The formation of nanodiamonds at near-ambient conditions confirms their remarkable stability and could help realize new technologies such as drug delivery and the coating of polymeric substrates. Gas-phase nucleation and in situ aerosol measurements The experimental set-up for the synthesis of nanodiamonds is schematically illustrated in Fig. 1a . This method has been previously applied to the synthesis of silicon nanoparticles with diameters <5 nm (ref. 17 ). To nucleate and grow carbon nanoparticles, mixtures of Ar and H 2 gas and ethanol vapour were continuously introduced and dissociated in the microplasma at atmospheric pressure and near-ambient neutral gas temperature ( Supplementary Fig. S1 ). Ethanol was chosen as the carbon precursor for several reasons. First, ethanol has been detected in interstellar gas and thus simulates a potential chemical environment for nanodiamond formation in outer space [18] . Second, the C:H:O ratio of ethanol is within the predicted composition range for solid carbon precipitation [19] and, by adding H 2 , the ratio can be systematically tuned from non-diamond to diamond phase growth. Finally, ethanol has a suitable vapour pressure, not too high, resulting in excessive soot formation, but not too low, preventing particle nucleation. When ethanol vapour was introduced into the microplasma, the discharge turned a bright blue-green colour as a result of C 2 emission (see Fig. 1a ). The neutral species gas temperature was estimated to be <100 °C using an infrared camera (FLIR, Inc.; Supplementary Fig. S2 ). The particles were collected at atmospheric pressure and room temperature by filtering the exiting aerosol flow with a fibre glass filter (see Fig. 1a ). Particle formation was monitored in situ by aerosol size classification using a commercial scanning mobility particle sizing (SMPS) system. 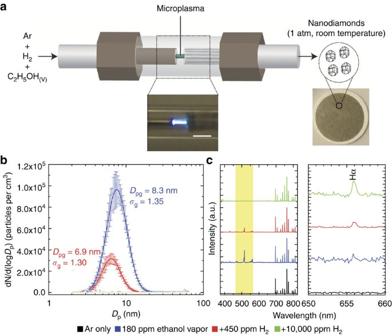Figure 1: Gas-phase nucleation andin situcharacterization of carbon nanoparticles. Carbon nanoparticles are synthesized in the gas phase by continuously dissociating a mixture of Ar, H2gas and ethanol vapour in an atmospheric pressure microplasma (a). Scale bar, 5 mm. The aerosol particles are collected as a dry product by filtration. Aerosol size classification confirms nanoparticle formation and shows that the addition of H2gas reduces the particle concentration and geometric mean diameter (Dpg). Error bars correspond to the standard error calculated from the geometric standard deviation (σg). Scale bar, 5mm. (b). Dissociation of ethanol vapour is monitored by OES (c). The C2band, which has been linked to nanodiamond formation, is clearly observed from 460 to 570 nm (left panel). The addition of H2gas results in the appearance of the HαBalmer line at 656 nm, confirming atomic hydrogen (right panel). Figure 1b shows particle size distributions (PSDs) for nanoparticles synthesized from 180 p.p.m. ethanol vapour in Ar and 180 p.p.m. ethanol vapour mixed with 450 and 10,000 p.p.m. H 2 gas in Ar. The PSDs represent an average of 10 scans collected by SMPS characterization after steady-state operation of the microplasma was reached. The raw data were fit to log-normal distributions to obtain the geometric mean diameters ( D pg ) and s.d. ( σ g ). We note that no particles were detected by the SMPS system for a pure Ar microplasma. The introduction of ethanol vapour produces a well-defined PSD, with a D pg of 8.3 nm at steady state. The addition of H 2 reduces the overall particle concentration and the D pg to 6.9 nm. Further increase in the gas-phase H 2 concentration to 10,000 p.p.m. completely quenches particle formation (see Fig. 1b ). These results are consistent with the C-H-O phase diagram for carbon growth that shows increasing H with respect to C in the gas phase eventually suppresses solid carbon nucleation [19] . Figure 1: Gas-phase nucleation and in situ characterization of carbon nanoparticles. Carbon nanoparticles are synthesized in the gas phase by continuously dissociating a mixture of Ar, H 2 gas and ethanol vapour in an atmospheric pressure microplasma ( a ). Scale bar, 5 mm. The aerosol particles are collected as a dry product by filtration. Aerosol size classification confirms nanoparticle formation and shows that the addition of H 2 gas reduces the particle concentration and geometric mean diameter ( D pg ). Error bars correspond to the standard error calculated from the geometric standard deviation ( σ g ). Scale bar, 5mm. ( b ). Dissociation of ethanol vapour is monitored by OES ( c ). The C 2 band, which has been linked to nanodiamond formation, is clearly observed from 460 to 570 nm (left panel). The addition of H 2 gas results in the appearance of the H α Balmer line at 656 nm, confirming atomic hydrogen (right panel). Full size image OES of precursor dissociation The dissociation of ethanol vapour and H 2 gas by the microplasma was confirmed by optical emission spectroscopy (OES). Figure 1c shows spectra collected from the microplasma for varying mixtures of Ar, ethanol vapour and H 2 gas. All spectra show evidence of lines corresponding to Ar 4p→4s transitions in the higher wavelength regions (665–815 nm) (ref. 20 ). When ethanol is introduced, additional peaks corresponding to the C 2 swan band between 460 and 570 nm (see left panel of Fig. 1c ) and CH modes at 387 and 431 nm are observed ( Supplementary Fig. S3a ). In addition, we detect excited H 2 from the Fulcher-α band system ~600 nm ( Supplementary Fig. S3b ) [20] . The confirmation of C 2 and CH radicals is particularly important for nanodiamond formation. Previous reports have shown that C 2 species initially nucleate a solid carbon cluster, and CH species form a hydrocarbon layer, promoting the nucleation of nanodiamonds [20] , [21] ; however, these experiments were carried out on films where the substrate may also influence nucleation [22] , [23] . The addition of H 2 gas results in a new feature in the OES spectra at 656 nm corresponding to the H α Balmer line (see right panel of Fig. 1c ). To quantify this observation, we compared the relative intensity of the H α line with an Ar-excited neutral line at 750.1 nm as a function of the gas-phase concentration of H 2 ( Supplementary Fig. S4 ). Increasing the H 2 gas concentration is found to increase the intensity of the H α line and decrease the H 2 band intensity, which indicates that dissociation to atomic hydrogen is a more favourable reaction channel than molecular excitation. The increase in atomic hydrogen coincides with a decrease in the particle diameter (see Fig. 1b ). Atomic hydrogen has been previously linked in CVD diamond growth to suppression of surface reconstruction [24] , etching of non-diamond (sp 2 ) carbon [20] , [25] and formation of surface radical sites by hydrogen abstraction [7] , suggesting that the smaller particle size corresponds to selective removal of the non-diamond phase and stabilization of the diamond phase in our as-grown material. Ultraviolet micro Raman spectroscopy The structure of the as-grown carbon nanoparticles was initially analysed by micro Raman spectroscopy. Ultraviolet (UV) excitation (325 nm) was employed to enhance the scattering from the sp 3 fraction in the samples [26] . Raman spectra are shown in Fig. 2a for carbon nanoparticles synthesized with only ethanol vapour (black) and a mixture of ethanol vapour and H 2 gas (red). Both spectra exhibit two broad features, one between 1,300 and 1,400 cm −1 and another at ~1,600 cm −1 , close to the D (disorder) and G (graphite) bands, respectively, which arise from K-point phonon scattering of A 1g symmetry and zone centre phonon scattering of E 2g symmetry, respectively, for sp 2 carbon materials. The first feature also overlaps with the well-known Raman scattering peak for bulk diamond at 1,332 cm −1 (ref. 26 ). The addition of H 2 gas is found to increase the peak intensity ratio of the first to the second feature, and shift the peak of the first feature to lower wavenumbers by ~40 cm −1 . A similar shift was also observed at other excitation wavelengths ( Supplementary Fig. S5 ). A small shift in the peak of the second feature from 1,593 to 1,603 cm −1 is also observed and maybe related to in-plane stretching of sp 2 carbon atoms resulting from strain introduced by the incorporation of hydrogen in the as-grown material. To further analyse the spectra, we deconvoluted and fit the features to Gaussian–Lorentzian curves ( Supplementary Table S1 ). As shown in the left inset of Fig. 2a , the spectrum for nanoparticles synthesized with only ethanol vapour consists of a peak at 1,397 cm −1 that can be assigned to a-C, and a weaker peak at 1,328 cm −1 . In comparison, the spectrum for nanoparticles synthesized with H 2 gas consists of two peaks at 1,307 and 1,372 cm −1 (right inset of Fig. 2a ), the former being significantly shifted to lower wavenumber and broadened. The confinement of optical phonons in nanodiamonds is known to cause a particle size-dependent shift to lower wavenumbers and broadening of the Raman scattering peak for bulk diamond [27] . Using a recently reported model [28] , we simulated Raman spectra as a function of nanodiamond particle size ( Supplementary Fig. S6 ). The calculated peak position and full width half maximum (FWHM) for 2.5-nm-diameter particles, 1,311 and 90 cm −1 ( Supplementary Table S2 and Supplementary Fig. S7 ), respectively, were found to agree well with our experimentally observed peak (1,307 cm −1 , FWHM=102 cm −1 ). We also obtained UV micro Raman spectra of commercial nanodiamond samples ( Supplementary Fig. S8a ). A similar analysis showed that the commercial samples primarily contain particles between 4 and 6 nm, larger than the particles found in our samples ( Supplementary Fig. S8b,c ). 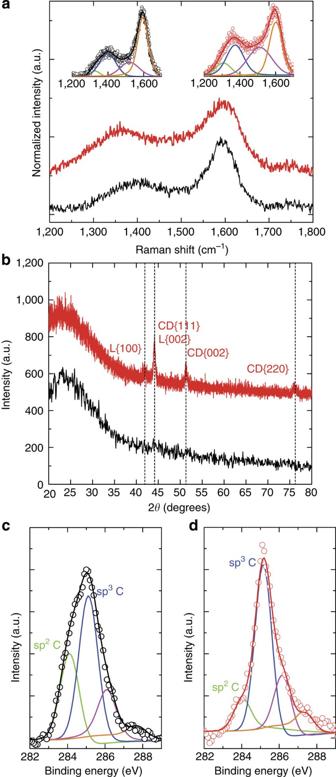Figure 2: Material characterization of carbon nanoparticles. (a) Micro Raman spectra of carbon nanoparticles synthesized with only ethanol vapour (black) and with ethanol vapour and H2gas (red). The addition of H2gas results in a shift of the broad feature near 1,400 cm−1to lower wavenumber. Deconvolution and fitting of this feature shows (inset ofa) evidence of a peak at 1,307 cm−1that agrees with phonon-confined scattering from nanodiamonds28. Excitation wavelength of 325 nm was used for all Raman spectra. (b) XRD patterns of carbon nanoparticles synthesized with only ethanol vapour (black) shows no crystalline peaks, suggesting an amorphous material. In comparison, the addition of H2gas results in crystalline peaks (red) that can be indexed to crystalline planes of lonsdaleite (L) and cubic diamond (CD) phases. (c,d)High-resolution C 1s XPS spectra of carbon nanoparticles synthesized with only ethanol vapour (c) and with ethanol vapour and H2gas (d). The different components corresponding to various chemical shifts of carbon bonds are indicated. The addition of H2gas increases the ratio of the sp3/sp2-hybridized carbon peak. Figure 2: Material characterization of carbon nanoparticles. ( a ) Micro Raman spectra of carbon nanoparticles synthesized with only ethanol vapour (black) and with ethanol vapour and H 2 gas (red). The addition of H 2 gas results in a shift of the broad feature near 1,400 cm −1 to lower wavenumber. Deconvolution and fitting of this feature shows (inset of a ) evidence of a peak at 1,307 cm −1 that agrees with phonon-confined scattering from nanodiamonds [28] . Excitation wavelength of 325 nm was used for all Raman spectra. ( b ) XRD patterns of carbon nanoparticles synthesized with only ethanol vapour (black) shows no crystalline peaks, suggesting an amorphous material. In comparison, the addition of H 2 gas results in crystalline peaks (red) that can be indexed to crystalline planes of lonsdaleite (L) and cubic diamond (CD) phases. ( c , d) High-resolution C 1s XPS spectra of carbon nanoparticles synthesized with only ethanol vapour ( c ) and with ethanol vapour and H 2 gas ( d ). The different components corresponding to various chemical shifts of carbon bonds are indicated. The addition of H 2 gas increases the ratio of the sp 3 /sp 2 -hybridized carbon peak. Full size image X-ray diffraction Figure 2b shows X-ray diffraction (XRD) patterns of the same two samples of carbon nanoparticles that were characterized by Raman spectroscopy. The XRD pattern for nanoparticles synthesized with only ethanol vapour (black) shows a broad peak at ~25°, indicating that the material is mostly a-C, consistent with Raman analysis. In comparison, carbon nanoparticles synthesized from a mixture of ethanol vapour and H 2 gas (red) exhibit clear diffraction peaks corresponding to lattice planes of various phases of diamond. A higher fraction of nanodiamonds in the sample grown with H 2 gas agrees with Raman analysis. The XRD peaks at 44.1°, 51.4° and 75.8° can be assigned to the (111), (002) and (220) lattice planes of cubic diamond, with a lattice parameter of 3.55 Å. We note that the (002) plane is a forbidden reflection for cubic diamond and corresponds to the n -diamond phase [29] . The stability of n -diamond is a point of contention, but its existence has been reported in both experiments [30] and theoretical calculations [31] . The structure of n -diamond is believed to be face-centered cubic, with hydrogen atoms incorporated into the cubic carbon lattice [30] . The formation of n -diamond is consistent with the increase in the concentration of atomic hydrogen with the addition of H 2 gas detected by OES. The peaks at 41.9° and 44.1°, the latter of which overlaps with cubic diamond, indicates the presence of lonsdaleite, with lattice constants of a =2.49 Å and c =4.11 Å (ref. 32 ). A mechanism for formation of lonsdaleite is not known, but this diamond phase is often found in meteorite samples [16] . In comparison, XRD patterns of commercial nanodiamond samples only showed the presence of the cubic phase ( Supplementary Fig. 9 ). We note that all XRD peak positions are slightly shifted towards higher 2 θ values as compared with bulk diamond, highlighting the nanoscale nature of our material and suggesting lattice compression due to surface stresses. X-ray photoelectron spectroscopy The purity of the diamond-phase in the as-synthesized carbon nanoparticles was assessed by X-ray photoelectron spectroscopy (XPS) [33] , [34] . From survey spectra, the metal content was found to be <0.1% in all samples ( Supplementary Table S3 and Supplementary Fig. S10 ). Figure 2c,d shows high-resolution C 1s XPS spectra collected from carbon nanoparticles synthesized with only ethanol vapour and a mixture of ethanol vapour and H 2 gas, respectively. XPS has been previously used to characterize the carbon bonding in a-C [33] , [35] and nanodiamond powders using C 1s spectra [34] , [36] , [37] . Although XPS is generally known to probe the surface of materials, for carbon materials the inelastic mean-free path of C 1s photoelectrons is ~3 nm. Thus, the whole volume of small nanoparticles, as in the case of our samples, was probed [34] . The C 1s signal of both samples consists of four chemically shifted components: peaks at ~284.0 and 285.0 eV corresponding to sp 2 - and sp 3 -hybridized carbon, respectively, and peaks at 286.1 and 287.4–287.7 eV corresponding to various hydrogen and oxygen functionalities including C-H, C-OH, C-O-C and C=O, in order of increasing binding energies. These peak shifts are in agreement with previous studies of nanodiamonds [34] , [37] . We focused our analysis on the sp 2 and sp 3 carbon peaks that arise from the presence of graphitic and diamond phases, respectively, in the samples. The sp 3 /sp 2 carbon ratio increases substantially from 1.6 to 5.5 with the addition of H 2 gas, corresponding to an increase in the fraction of sp 3 carbon relative to sp 2 carbon from ~61 to 85% ( Supplementary Table S4 ). We validated the reliability of XPS to assess the purity of the diamond phase with respect to the graphitic phase by also characterizing several commercially available nanodiamond samples and found excellent agreement with reported values ( Supplementary Fig. S11 ) [38] . Overall, our XPS results confirm that the addition of H 2 gas improves the as-synthesized purity of the nanodiamonds relative to non-diamond carbon. Although atomic hydrogen has been previously used to treat nanodiamond powder and remove sp 2 carbon [39] , the key difference is that in our process the nanodiamonds are purified in flight. Transmission electron microscopy Additional microstructural characterization of our material was performed at the nanoscale by transmission electron microscopy (TEM). 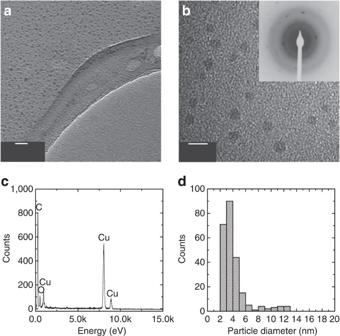Figure 3: TEM analysis of carbon nanoparticles. Representative TEM image of as-grown carbon nanoparticles synthesized by dissociation of only ethanol vapour in an atmospheric pressure microplasma shows evidence of unagglomerated, nanosized particles (a). The particles are roughly spherical and highly uniform in size. Scale bar, 20 nm. (b). SAED confirms that the particles are crystalline (inset ofb). EDX shows that the particles are metal-free (Cu peaks are from the TEM grid). Scale bar, 5 nm (c). Histogram of the particle diameters as measured from TEM analysis of ~250 particles shows that the particles are primarily between 2 and 5 nm (d). Figure 3a,b shows representative TEM images of carbon nanoparticles synthesized from only ethanol vapour and drop-cast on carbon-coated Cu grids from a solution dispersion. The nanoparticles are unagglomerated ( Fig. 3a ), uniformly sized ( Fig. 3b ) and crystalline, as confirmed by selected-area electron diffraction (SAED; inset of Fig. 3b ). The chemical composition of the particles was assessed by energy-dispersive spectroscopy (EDX). The EDX spectrum in Fig. 3c shows that the particles are free of impurities, in support of XPS results; peaks in the spectra from copper and oxygen are always present from the Cu grid and O 2 gas in the instrument background. A histogram obtained by sizing and counting ~250 individual particles from TEM images shows that the nanoparticles are mostly between 2 and 5 nm diameter (>90%). The monodispersity of the particles supports the existence of a ‘magic’ cluster size [15] . 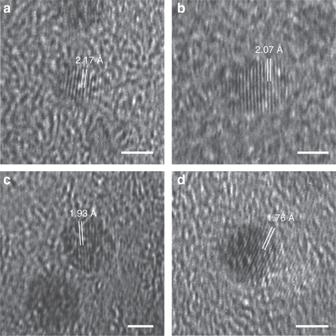Figure 4: High-resolution TEM of nanodiamonds. Measured lattice spacings of single particles correspond to the lonsdaleite (100) (a), cubic diamond (111) or lonsdaleite (002) (b), lonsdaleite (101) (c), and cubic diamond (002) (d) phases. Scale bars, 2 nm. Figure 4 shows high-resolution TEM analysis of individual particles whose random orientation allowed lattice fringes to be observed. The measured lattice spacings match up well with lattice planes of various diamond phases including lonsdaleite (100) (2.17 Å), cubic diamond (111) or lonsdaleite (002) (2.07 Å), lonsdaleite (101) (1.93 Å) and cubic diamond (002) (1.76 Å). The latter suggests the presence of the previously described n -diamond phase. We performed similar single-particle lattice spacing measurements on ~50 particles and combined this analysis with SAED and XRD to statistically assess the crystal structure of the nanodiamonds in our samples ( Supplementary Table S5 and Supplementary Figs S12–S16 ). Table 1 summarizes the measured d spacings, all of which within error compare favourably with reported values for cubic diamond, n -diamond and lonsdaleite [2] , [40] . Figure 3: TEM analysis of carbon nanoparticles. Representative TEM image of as-grown carbon nanoparticles synthesized by dissociation of only ethanol vapour in an atmospheric pressure microplasma shows evidence of unagglomerated, nanosized particles ( a ). The particles are roughly spherical and highly uniform in size. Scale bar, 20 nm. ( b ). SAED confirms that the particles are crystalline (inset of b ). EDX shows that the particles are metal-free (Cu peaks are from the TEM grid). Scale bar, 5 nm ( c ). Histogram of the particle diameters as measured from TEM analysis of ~250 particles shows that the particles are primarily between 2 and 5 nm ( d ). Full size image Figure 4: High-resolution TEM of nanodiamonds. Measured lattice spacings of single particles correspond to the lonsdaleite (100) ( a ), cubic diamond (111) or lonsdaleite (002) ( b ), lonsdaleite (101) ( c ), and cubic diamond (002) ( d ) phases. Scale bars, 2 nm. Full size image Table 1 Crystal structure analysis. Full size table A small number of particles were appropriately oriented with the electron beam in TEM to allow more than one crystal plane of individual particles to be resolved. 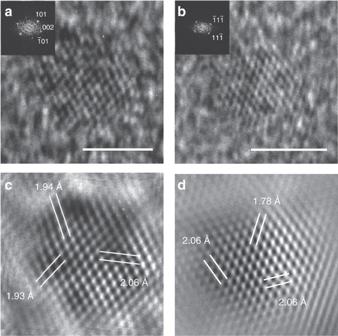Figure 5: Single-particle analysis by FFT filtering. (a,b) High-resolution transmission electron microscopy images of two nanodiamond particles aligned with the electron beam and imaged along the (010) (a) and (110) (b) zone axes. Corresponding FFT images (insets ofa,b) and inverse FFT images (c,d) confirm that the particles are lonsdaleite (a,c) andn-diamond (b,d), respectively. Scale bars, 2 nm. Figure 5a,b shows high-resolution transmission electron microscopy images of two representative particles, both 3 nm in diameter. From the fast Fourier transform images (FFT; see insets of Fig. 5a ), we determined that the particles are lonsdaleite and n -diamond, imaged along the (010) and (110) zone axes, respectively. The measured lattice spacings from the corresponding inverse FFT images shown in Fig. 5c,d validate the crystalline structure and are in excellent agreement with SAED and XRD results (see Table 1 ). Figure 5: Single-particle analysis by FFT filtering. ( a , b ) High-resolution transmission electron microscopy images of two nanodiamond particles aligned with the electron beam and imaged along the (010) ( a ) and (110) ( b ) zone axes. Corresponding FFT images (insets of a , b ) and inverse FFT images ( c , d ) confirm that the particles are lonsdaleite ( a , c ) and n -diamond ( b , d ), respectively. Scale bars, 2 nm. Full size image Carbon nanoparticles synthesized by adding H 2 gas to the ethanol vapour in the microplasma were also analysed by TEM ( Supplementary Fig. S17 ). In comparison with carbon nanoparticles synthesized with only ethanol vapour, we observed that the samples were much cleaner (less a-C), consistent with micro Raman, XRD and XPS characterization. The particles were unagglomerated and crystalline, with similar particle sizes and crystal structures as those synthesized with only ethanol vapour ( Supplementary Fig. S18 ). Commercial nanodiamond samples imaged by TEM were found to be comparatively larger in size (>5 nm), in agreement with Raman characterization, and severely agglomerated ( Supplementary Fig. S19 ). There are several possible reasons why our process is capable of producing nanodiamonds at near-ambient conditions. The microplasma process is comparable to PECVD and the combination of plasma dissociation and gas-phase chemistry may aid the nucleation of diamond-phase carbon analogous to chemical vapour deposition (CVD) diamond [19] . Similar to CVD, atomic hydrogen may kinetically etch the non-diamond sp 2 carbon and allow diamond-phase sp 3 carbon to grow [1] . Hydrogen may also help stabilize the surface of the nanodiamonds [3] . Previous attempts to synthesize carbon nanoparticles by homogeneous nucleation have produced graphene [12] or much larger diamond particles [14] . The formation of nanodiamonds in a microplasma underscores the importance of quenching, which maybe essential to limiting the particle size to diamond’s predicted thermodynamic stability at the nanoscale [3] . Future studies are required to more carefully clarify the mechanism for nanodiamond formation in our process and, in particular, separate these kinetic and thermodynamic considerations. The formation of nanodiamonds at near-ambient conditions has wide-ranging scientific implications. Our experimental confirmation of diamond-phase carbon produced at conditions far from its bulk thermodynamic stability provides support for theoretical predictions, and, importantly, the size at which this occurs ( ca. 3 nm) [3] . The ‘magic’ size [15] and structure of the material, including the more rare lonsdaleite phase, is consistent with characterization of interstellar diamond [16] and suggests that a high-pressure history is not needed to explain their existence [41] . The evidence for gas-phase nucleation in a plasma environment brings into question how diamond maybe nucleated in conventional CVD processes [9] and suggests that diamond particles could in some cases nucleate first in the gas phase, subsequently deposit on the substrate and act as seeds for film growth. The process we have developed should also have several technological benefits. Compared with CVD, nanodiamonds are synthesized continuously at atmospheric pressure and as a powder. By fabricating arrays of microplasmas, it should be possible to produce large mass amounts (>1 g h −1 ) [42] . The nanodiamonds are produced at significantly lower temperatures, which should enable the coating of plastics for flexible applications [43] . Compared with detonation, the microplasma process is higher purity as metal and other impurities (for example, nitrogen and oxygen) are eliminated [44] . Moreover, steep pressure and temperature gradients are avoided, which in detonation processes lead to fullerene shells and severe agglomeration, requiring extensive post-purification steps [45] . Through the addition of H 2 gas, we have shown a path to improve the purity of the diamond phase in flight, as opposed to acid treatment [45] and air oxidation [38] . Finally, our results indicate that the nanodiamonds produced by the microplasma process are significantly smaller than currently available material [10] . Such particles may facilitate biological applications where the particle size is critical to transport and drug delivery [46] . Overall, these differences suggest that it maybe possible through future studies to further tune and optimize the microplasma process to ultimately control the particle size, surface chemistry and doping (for example, nitrogen) of the nanodiamonds for a wide range of applications. Microplasma synthesis and aerosol mobility measurements Carbon nanoparticles were synthesized in the gas phase at atmospheric pressure and room temperature by continuously dissociating ethanol vapour in a microplasma. The microplasma was formed between a stainless steel capillary tube (outer diameter=1.59 mm, inner diameter=0.178 mm) and a stainless steel mesh (2 × 4 mm 2 ) electrode, operated as the cathode and anode, respectively. The electrodes were separated by a gap of 2 mm and sealed inside a quartz tube (OD=6.35 mm) with Swagelok gas fittings. The microplasma was ignited with a negatively biased, high-voltage, direct-current power supply (Power Designs Inc, Model HV-1547), ballasted by a power resistor (500 kΩ). The discharge was operated at a constant current of 3.6 mA in all experiments. Controlled concentrations of ethanol vapour were introduced into the microplasma by bubbling Ar gas through a solution of pure ethanol (200 proof, Decon Labs, Inc.) cooled to −10 °C (* P =0.1079, psi, 5,000 p.p.m.). This flow was then diluted twice, first with a flow of 460 s.c.c.m. Ar, and then with a flow of 55 s.c.c.m. Ar after exhausting a flow of 455 s.c.c.m. Thus, a final concentration of 180 p.p.m. ethanol in Ar at a total gas flow rate of 100 s.c.c.m. was introduced into the microplasma. From aerosol measurements, we found that this ethanol concentration was optimal to nucleate a steady-state concentration of carbon nanoparticles for over 100 h. Alternatively, we introduced H 2 gas either directly into the microplasma at a concentration of 10,000 p.p.m. or with Ar through the bubbler for a final H 2 concentration of 450–1,800 p.p.m. in the microplasma. In situ aerosol measurements of as-synthesized carbon nanoparticles were performed with a scanning mobility particle sizer (SMPS) system (TSI, Inc., Model 3936) consisting of a differential mobility analyser and a butanol-based condensation particle counter. To avoid Brownian coagulation, the particles exiting the microplasma were diluted with a flow of N 2 gas. Optical emission spectroscopy OES of the microplasma was carried out by collecting the emitted light with a 600-μm-diameter fibre optic cable coupled to a spectrometer (Ocean Optics Inc., Model HR400). Line intensities were calibrated with a tungsten halogen light source. Spectra were integrated 10 times with an acquisition time of 100 ms. Collection of carbon nanoparticles As-synthesized carbon nanoparticles were collected by continuously trapping the aerosol product exiting the microplasma on commercial filters with pore sizes <1 μm including stainless steel, polyfluorotetraethylene and glass fibre. In most cases, we used glass fibre filters (Millipore Inc.) that did not contribute any background signal in micro Raman spectroscopy and XRD. The mass of collected product was obtained by weighing the filter before and after collection. Micro Raman spectroscopy and phonon confinement model Micro Raman spectroscopy was carried out at various excitation wavelengths. Excitation in the visible range was performed with an inVia Renishaw spectrometer equipped with three lasers at λ =488, 514 and 633 nm. To enhance the scattering from the sp 3 component relative to the sp 2 component of our material [26] , UV excitation at λ =325 nm was performed with a Jobin-Yvon LabRAM HR800 spectrometer. The Raman spectra were fit to a refined phonon confinement model [28] for diamond, which relates the intensity of the Raman scattering to the size of the particles: where I is the intensity, L is the size of the particles, ω is the phonon dispersion curve, q is the wave vector and Γ is the FWHM of the scattering peak. Γ and ω ( q ) are given by the following polynomial functions: where A =11 cm −1 and B =491.25 cm −1 and where A , B , C , D , E and F are coefficients for seven different phonon branches (Λ 1 , Λ 3, Σ 1 , Σ 2, Σ 3, Δ 2 and Δ 5 ) corresponding to scattering from various crystalline phases of diamond. XRD XRD was carried out with a Scintag X-1 advanced X-ray diffractometer using monochromated Cu-Kα radiation ( λ =0.1542, nm). All XRD patterns were collected from a 2 θ of 20°–80°, with a step size of 0.01°, at a grazing incident angle of 2° to enhance the sensitivity from our relatively thin samples. From the XRD peaks, d spacings were calculated using Bragg’s equation ( n λ=2dsinθ). For d spacings corresponding to cubic or n -diamond, the lattice parameter, a , was calculated using the following equation: and for d spacings corresponding to the lonsdaleite phase of diamond, the lattice parameters, a and c were calculated using the following equation (where a = b ≠ c ): XPS XPS was performed with a PHI VersaProbe using a monochromatic Al Kα X-ray (1486.6 eV) source. Samples for XPS were either prepared by collecting on glass fibre filters to assess the metal impurities or directly depositing on single crystal Si substrates using a nanometre aerosol sampler (TSI, Inc., Model 3089) to characterize the relative fraction of diamond (sp 3 carbon) and non-diamond (sp 2 carbon) phases. Before nanoparticle deposition, the Si substrates were cleaned with acetone to remove residual carbon. After deposition, the samples were sputtered inside the XPS instrument by an Ar ion beam to remove contamination (for example, adventitious carbon) that occurred during sample transfer. In all cases, spectra were taken with a spot size of 300 μm. High-resolution C 1s spectra were acquired with a step size of 0.1 eV from a minimum of two spots on each sample and averaged. The binding energies were corrected to compensate for surface charging. The spectra were deconvoluted and fit using the PHI Multipak program from ULVAC-PHI, Inc. by a Lorentz−Gauss algorithm after subtracting a Shirley background. TEM and EDX TEM was carried out with a Philips Tecnai F30 field-emission electron microscope operated at 300 kV. TEM samples were prepared by carefully shaking the filter-collected carbon nanoparticles in methanol and drop casting on carbon-coated Cu grids. Sonication was avoided to prevent the filter from breaking up. EDX was performed with a 130-eV energy resolution Li-drift Si detector. Additional structural information was obtained by SAED and FFT. How to cite this article: Kumar, A. et al . Formation of nanodiamonds at near-ambient conditions via microplasma dissociation of ethanol vapour. Nat. Commun. 4:2618 doi: 10.1038/ncomms3618 (2013).